Activation of canonical Wnt signalling is required for TGF-β-mediated fibrosis The transforming growth factor-β (TGF-β) signalling pathway is a key mediator of fibroblast activation that drives the aberrant synthesis of extracellular matrix in fibrotic diseases. Here we demonstrate a novel link between transforming growth factor-β and the canonical Wnt pathway. TGF-β stimulates canonical Wnt signalling in a p38-dependent manner by decreasing the expression of the Wnt antagonist Dickkopf-1. Tissue samples from human fibrotic diseases show enhanced expression of Wnt proteins and decreased expression of Dickkopf-1. Activation of the canonical Wnt pathway stimulates fibroblasts in vitro and induces fibrosis in vivo . Transgenic overexpression of Dickkopf-1 ameliorates skin fibrosis induced by constitutively active TGF-β receptor type I signalling and also prevents fibrosis in other TGF-β-dependent animal models. These findings demonstrate that canonical Wnt signalling is necessary for TGF-β-mediated fibrosis and highlight a key role for the interaction of both pathways in the pathogenesis of fibrotic diseases. Activation of fibroblasts and their differentiation into myofibroblasts with increased release of extracellular matrix proteins is a key feature of fibrotic diseases. The extracellular matrix accumulates and disrupts the physiological tissue architecture [1] . Tissue fibrosis may occur after defined stimuli, but in many cases, no initiating trigger can be identified. These idiopathic fibrotic diseases can affect virtually every organ system. Fibrosis may be restricted to single organs such as the lungs or the liver or manifest as systemic fibrotic disease involving multiple organ systems. Systemic sclerosis (SSc) is a prototypical idiopathic systemic fibrotic disease that affects the skin and several internal organs such as lungs, heart, gastrointestinal tract and kidneys [2] . Similar to other fibrotic diseases, failure of the affected organs is common and results in high morbidity and significantly increased mortality. The molecular mechanisms leading to aberrant activation of fibroblasts and persistently increased release of extracellular matrix components are incompletely understood, and molecular therapies for the treatment of fibrosis are not yet available for clinical use [3] . There is considerable evidence that transforming growth factor-β (TGF-β) is a key regulator of fibroblast activation in fibrotic diseases [4] , [5] . The levels of TGF-β are elevated in fibrotic diseases and fibroblasts display activation of TGF-β signalling with nuclear accumulation of active Smad3 and increased transcription of TGF-β target genes [6] . Moreover, TGF-β induces a gene expression profile in resting fibroblasts that is reminiscent of activated fibroblasts [7] . The central role of TGF-β signalling is further highlighted by the development of a systemic fibrotic disease in mice with fibroblast-specific overexpression of constitutively active TGF-β receptor type I (ref. 8 ). The effects of TGF-β are mediated by a complex network of intracellular signalling events. Evolutionarily conserved Smad proteins are considered as major signalling intermediaries for the stimulatory effects of TGF-β in fibroblasts [9] . Smad-independent signal transducers such as mitogen-activated protein kinases, focal adhesion kinase, the tyrosine kinase c-ABL and early growth response 1 have also been implicated in the profibrotic effects of TGF-β [5] . However, inhibition of these downstream pathways does not completely abrogate the stimulatory effects of TGF-β on fibroblasts, indicating that additional pathways are important for transmission of the profibrotic effects of TGF-β. Identification of these novel downstream mediators of TGF-β might have direct translational implications. Wnt signalling profoundly affects developmental processes during embryogenesis and has an important role for tissue homeostasis in adults [10] , [11] . Wnt proteins are secreted ligands that transmit their signal across the plasma membrane by interacting with Frizzled receptors and low-density lipoprotein receptor-related protein co-receptors (LRP5/6) (refs 12 , 13 ). Upon binding to their receptors, Wnt proteins induce a cascade of intracellular signalling events, involving proteins such as Disheveled, Axin, Adenomatosis Polyposis Coli and Glycogen Synthase Kinase-3β, that culminates in the stabilization of β-catenin. β-catenin translocates to the nucleus, where it binds to T-cell factor/lymphoid enhancer-binding factor (Tcf/Lef) to induce the transcription of Wnt target genes [14] . In addition to this canonical pathway, certain Wnt proteins exert their effects by activation of the planar cell polarity pathway and the calcium/calmodulin-dependent kinase pathway [15] . Aberrant activation of the canonical Wnt pathway either by mutations of intracellular regulators or by altered expression of Wnt proteins or endogenous inhibitors of Wnt signalling has been implicated in a variety of different diseases [16] , [17] . Of particular interest, accumulating evidence indicates that increased activation of canonical Wnt signalling might have an important role in fibrogenesis. So far, pathologically activated canonical Wnt has been implicated in the pathogenesis of pulmonary-, renal-, dermal- and liver fibrosis as well as in scarring after myocardial fibrosis and fibrosis following muscular dystrophy [18] , [19] , [20] , [21] , [22] , [23] , [24] , [25] , [26] , [27] . To avoid uncontrolled activation, canonical Wnt signalling is tightly controlled by an array of negative regulators. Among those, Dickkopf proteins (Dkk-1–4) seem to have a key role. The best studied member is Dkk-1, which functions as a natural secreted antagonist of Wnt signalling [28] , [29] . Two different mechanisms have been suggested by which Dkk-1 inhibits canonical Wnt signalling. The first model proposes that Dkk-1 binds to LPR5/6 and its co-receptor Kremen-1/2, which promotes internalization of the receptor complex and degradation of LRPs. However, more recent studies suggest that the inhibitory effect of Dkk-1 is more likely mediated by disruption of the ternary complex between Wnt, LRP5/6 and Frizzled receptors, and that Kremen-1/2 are not universally required for Dkk-1 function, but rather have a modulatory function in certain tissues [30] , [31] . In this study, we show that the canonical Wnt pathway is activated in fibrotic diseases and potently stimulates fibroblast activation and tissue fibrosis. TGF-β signalling decreases the expression of Dkk-1 and activates the Wnt pathway. Inhibition of canonical Wnt signalling by overexpression of Dkk-1 potently reduces the profibrotic effects of TGF-β, demonstrating that the interaction of the canonical Wnt pathway and TGF-β has a key role in the pathogenesis of fibrotic diseases. Activation of the canonical Wnt pathway in fibrosis To investigate the activation of the canonical Wnt cascade, we first assessed the nuclear accumulation of β-catenin in human fibrotic tissue. Skin sections derived from patients with SSc were triple stained for β-catenin, the fibroblast marker prolyl-4-hydroxylase-β and 4,6-diamidino-2-phenylindole (DAPI). Nuclear β-catenin was detected in more than 80% of fibroblasts as compared with 25% of fibroblasts in the skin of healthy individuals ( Fig. 1a and Supplementary Fig. S1 ). The results were additionally confirmed by triple staining for vimentin, another fibroblast marker, β-catenin and DAPI. A prominent activation of the canonical Wnt pathway in fibroblasts with nuclear accumulation of β-catenin was also observed in idiopathic pulmonary fibrosis and liver cirrhosis ( Fig. 1a ), suggesting that activation of the canonical Wnt pathway is a general feature of human fibrotic disease. The canonical Wnt pathway was also activated in different experimental models of fibrosis with increased nuclear accumulation of β-catenin in bleomycin-induced dermal fibrosis and in tight-skin-1 (Tsk-1) mice ( Fig. 1a ). Consistent with the increased nuclear accumulation of β-catenin, the mRNA levels of axin-2, a classical target of the canonical Wnt pathway, were significantly increased in human fibrotic disease and in murine experimental fibrosis ( Fig. 1b ). 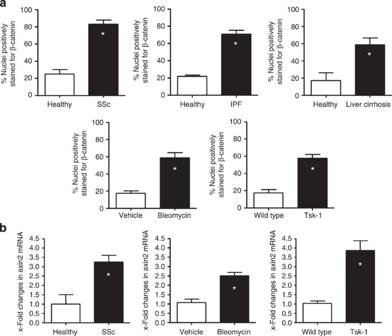Figure 1: Canonical Wnt signalling is activated in fibrotic diseases. (a) β-catenin, the central signalling component of the canonical Wnt pathway, accumulated in the nuclei of fibroblasts in samples from patients with SSc (n=12 for SSc andn=10 for normal skin), IPF (n=8 for IPF andn=6 for non-fibrotic lung) and liver cirrhosis (n=6 for liver cirrhosis andn=6 for non-fibrotic liver). Nuclear accumulation of β-catenin in dermal fibroblasts was also observed in the experimental models of bleomycin-induced dermal fibrosis and in Tsk-1 mice (n=10 each). A minimum of 100 nuclei per sample was counted. (b) The mRNA levels of the Wnt target gene axin-2 were significantly increased in systemic sclerosis patients, bleomycin challenged mice and Tsk-1 mice (n=8 each). * IndicatesP-values of less than 0.05 (analysed using the Mann–WhitneyU-test) as compared with healthy volunteers or with non-fibrotic control mice, respectively. All data are expressed as mean ± s.e.m. Figure 1: Canonical Wnt signalling is activated in fibrotic diseases. ( a ) β-catenin, the central signalling component of the canonical Wnt pathway, accumulated in the nuclei of fibroblasts in samples from patients with SSc ( n =12 for SSc and n =10 for normal skin), IPF ( n =8 for IPF and n =6 for non-fibrotic lung) and liver cirrhosis ( n =6 for liver cirrhosis and n =6 for non-fibrotic liver). Nuclear accumulation of β-catenin in dermal fibroblasts was also observed in the experimental models of bleomycin-induced dermal fibrosis and in Tsk-1 mice ( n =10 each). A minimum of 100 nuclei per sample was counted. ( b ) The mRNA levels of the Wnt target gene axin-2 were significantly increased in systemic sclerosis patients, bleomycin challenged mice and Tsk-1 mice ( n =8 each). * Indicates P -values of less than 0.05 (analysed using the Mann–Whitney U -test) as compared with healthy volunteers or with non-fibrotic control mice, respectively. All data are expressed as mean ± s.e.m. Full size image Searching for Wnt family members that might stimulate the activation of the canonical Wnt cascade, we found an overexpression of Wnt-1 and Wnt-10b in human fibrotic diseases. Wnt-1 and Wnt-10b were strongly expressed in fibrotic skin from patients with SSc ( Fig. 2a and b ). In contrast, in non-fibrotic skin, Wnt-1 was almost undetectable and the expression of Wnt-10b was reduced, in particular, in the dermal compartment ( Fig. 2a ). The overexpression of Wnt-1 and Wnt-10b was not restricted to fibrotic skin, but was also observed in pulmonary fibrosis and liver cirrhosis ( Fig. 2a and b ). Costaining with the fibroblast markers prolyl-4-hydroxylase-β or vimentin demonstrated that fibroblasts were a major source of Wnt-1 and Wnt-10b. However, the expression of Wnt proteins is not restricted to fibroblasts, but is also found in other cell types ( Fig. 2a and b ). Wnt-2b-13, Wnt-3a, Wnt-6, Wnt-7a, Wnt-7b and Wnt-8a were not detectable in all samples by real-time PCR. mRNA for Wnt-2, Wnt-9a, Wnt-9b and Wnt-16 was detected only in few samples without differences between SSc patients and controls. Wnt-4 mRNA was detected in the majority of fibrotic skin samples, no differences in the intensity or the expression pattern of Wnt-4 protein were observed between fibrotic skin and controls by immunohistochemistry. 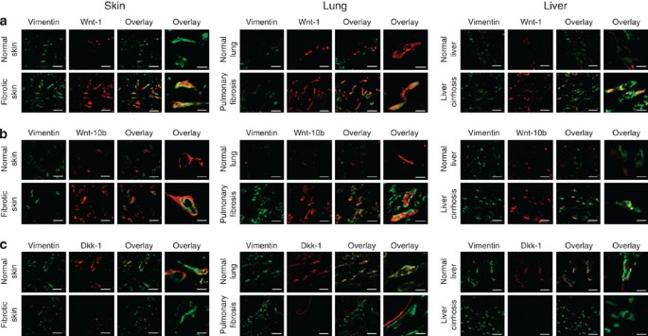Figure 2: Wnt-1 and Wnt-10b are upregulated in fibrotic diseases and Dkk-1 is downregulated. (a) Confocal microscopy with double staining for Wnt-1 and vimentin demonstrated an overexpression of Wnt-1, in particular, in vimentin-positive cells in fibrotic skin of patients with SSc, in IPF and in liver cirrhosis. (b) Wnt-10b was also overexpressed in SSc, IPF and liver cirrhosis. (c) In parallel to the upregulation of Wnt-1 and Wnt-10b, a prominent decrease of the endogenous antagonist Dkk-1 was observed in fibroblasts in fibrotic diseases. Representative examples from 12 patients with SSc, 10 samples of non-fibrotic skin, 10 patients with IPF, 6 control lungs, 8 patients with liver cirrhosis and 8 control livers are shown. Scale bars, 20 or 5 μm for the outer right image of each panel, respectively. Figure 2: Wnt-1 and Wnt-10b are upregulated in fibrotic diseases and Dkk-1 is downregulated. ( a ) Confocal microscopy with double staining for Wnt-1 and vimentin demonstrated an overexpression of Wnt-1, in particular, in vimentin-positive cells in fibrotic skin of patients with SSc, in IPF and in liver cirrhosis. ( b ) Wnt-10b was also overexpressed in SSc, IPF and liver cirrhosis. ( c ) In parallel to the upregulation of Wnt-1 and Wnt-10b, a prominent decrease of the endogenous antagonist Dkk-1 was observed in fibroblasts in fibrotic diseases. Representative examples from 12 patients with SSc, 10 samples of non-fibrotic skin, 10 patients with IPF, 6 control lungs, 8 patients with liver cirrhosis and 8 control livers are shown. Scale bars, 20 or 5 μm for the outer right image of each panel, respectively. Full size image In addition to the upregulation of Wnt-1 and Wnt-10b, the expression of the endogenous inhibitor Dkk-1 was strongly decreased in fibrotic diseases ( Fig. 2c ). Fibroblasts in non-fibrotic skin expressed Dkk-1, whereas the expression of Dkk-1 was virtually absent in fibroblasts in fibrotic skin. The expression of Dkk-1 was also decreased in pulmonary fibrosis and in liver cirrhosis compared with non-fibrotic lung and liver ( Fig. 2c ). We also analysed the levels of other inhibitors of Wnt signalling. sFRP3, sFRP4, sFRP5, Dkk-3, Dkk-4 and DkkL-1 were undetectable by real-time PCR. Expression of sFRP1, sFRP2 or Dkk-2 mRNA was detected in skin samples, but no differences were observed between fibrotic tissue and controls. Canonical Wnt signalling induces fibrosis To investigate the functional role of the canonical Wnt pathway in fibrosis, human dermal fibroblasts were incubated with Wnt-1, which we found upregulated in human fibrotic diseases. Wnt-1 stimulated the transcriptional activity in Col1a2 reporter assays ( Fig. 3a ). The increase in promoter activity on simultaneous stimulation with TGF-β and Wnt-1 was only slightly higher than with single stimulation with TGF-β or Wnt-1. Consistently, a dose-dependent increase in collagen release was observed in the supernatants of fibroblasts stimulated with Wnt-1 ( Fig. 3b ). Of note, the stimulatory effects of Wnt-1 were comparable with those of TGF-β, which is considered to belong to the most potent profibrotic mediators. Next, we analysed whether the increased release of collagen on stimulation with Wnt-1 might result from increased differentiation of resting fibroblasts into myofibroblasts. Myofibroblasts produce large amounts of extracellular matrix and have a key role in fibrotic diseases [2] . Incubation of resting fibroblasts with Wnt-1 increased the levels of α-smooth muscle actin (αSMA) protein and mRNA ( Fig. 3c and d ) and induced the formation of stress fibres ( Fig. 3e ), demonstrating increased differentiation of resting fibroblasts into myofibroblasts. In addition to Wnt-1, other Wnt proteins such as Wnt-3a also stimulated the release of collagen and induced differentiation of resting fibroblasts into myofibroblasts. 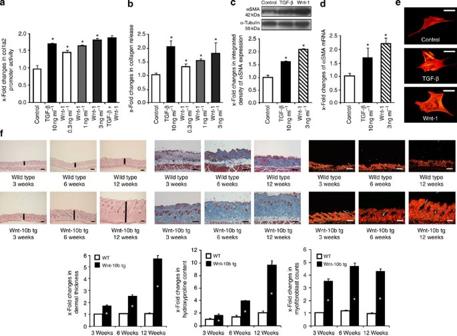Figure 3: Activation of the canonical Wnt pathway induces fibrosis. (a) Recombinant Wnt-1 stimulated the activity of col1a2 promoter constructs (n=6). (b) Incubation with recombinant Wnt-1 increased the release of collagen protein by cultured fibroblasts in a dose-dependent manner (n=6). (c) Wnt-1 induced the expression of αSMA protein (n=5). (d) Incubation with Wnt-1 increased the mRNA levels of αSMA (n=5). (e) Wnt-1 stimulated the formation of stress fibres in cultured fibroblasts (n=6). Of note, the stimulatory effects of Wnt-1 on fibroblasts were comparable with those of TGF-β. (f) Transgenic overexpression of Wnt-10b induced dermal fibrosis in mice. The dermal thickness, the hydroxyproline content and the numbers of myofibroblasts were already increased in Wnt-10b tg mice at an age of 3 weeks and increased further with age (n≥ 5 for all groups). Representative haematoxylin and eosin-, trichrome- and Sirius Red-stained sections of wild-type (WT) and Wnt-10b transgenic (Wnt-10b tg) mice at ages of 3, 6 and 12 weeks are shown (horizontal scale bars, 100 μm). Black vertical bars indicate the dermal thickness. * IndicatesP-values of less than 0.05 as compared with mock-treated fibroblasts (a–e, analysed with the Wilcoxon signed-rank test) or compared with wild-type littermates (f, analysed using the Mann–WhitneyU-test), respectively. All data are expressed as mean ± s.e.m. Figure 3: Activation of the canonical Wnt pathway induces fibrosis. ( a ) Recombinant Wnt-1 stimulated the activity of col1a2 promoter constructs ( n =6). ( b ) Incubation with recombinant Wnt-1 increased the release of collagen protein by cultured fibroblasts in a dose-dependent manner ( n =6). ( c ) Wnt-1 induced the expression of αSMA protein ( n =5). ( d ) Incubation with Wnt-1 increased the mRNA levels of αSMA ( n =5). ( e ) Wnt-1 stimulated the formation of stress fibres in cultured fibroblasts ( n =6). Of note, the stimulatory effects of Wnt-1 on fibroblasts were comparable with those of TGF-β. ( f ) Transgenic overexpression of Wnt-10b induced dermal fibrosis in mice. The dermal thickness, the hydroxyproline content and the numbers of myofibroblasts were already increased in Wnt-10b tg mice at an age of 3 weeks and increased further with age ( n ≥ 5 for all groups). Representative haematoxylin and eosin-, trichrome- and Sirius Red-stained sections of wild-type (WT) and Wnt-10b transgenic (Wnt-10b tg) mice at ages of 3, 6 and 12 weeks are shown (horizontal scale bars, 100 μm). Black vertical bars indicate the dermal thickness. * Indicates P -values of less than 0.05 as compared with mock-treated fibroblasts ( a – e , analysed with the Wilcoxon signed-rank test) or compared with wild-type littermates ( f , analysed using the Mann–Whitney U -test), respectively. All data are expressed as mean ± s.e.m. Full size image We next investigated whether the stimulatory effects of Wnts on fibroblasts result from direct TCF binding to collagen and αSMA promoters or are mediated indirectly by other Wnt target genes. Maximal increases of col1a2 reporter activity, collagen and αSMA mRNA levels occurred as late as 24 h after stimulation with Wnt proteins. The corresponding increases on the protein level were maximal after 48 h. The delayed induction indicates an indirect mechanism rather than a direct, TCF-mediated effect. Indeed, promoter analysis of 10,000 bp upstream of the col1a1 and col1a2 gene did not identify TCF binding elements. To confirm these findings, the effect of recombinant Wnt-1 on the synthesis of collagen was measured in the presence of cycloheximide, an inhibitor of translation. Cycloheximide completely blocked the induction of col1a1 mRNA, demonstrating that the stimulatory effects of Wnt-1 on collagen synthesis are indirect and require protein neosynthesis ( Supplementary Fig. S2 ). Having demonstrated that the canonical Wnt cascade stimulates the release of collagen and myofibroblast differentiation in vitro , we next used Wnt-10b transgenic (tg) mice to investigate whether activation of the canonical Wnt pathway is sufficient to induce fibrosis in vivo . Activation of canonical Wnt signalling in dermal fibroblasts in Wnt-10b tg mice was confirmed by demonstration of nuclear accumulation of β-catenin ( Supplementary Fig. S3 ) and increased mRNA levels of the target gene axin-2. Transgenic overexpression of Wnt-10b resulted in a massive generalized dermal fibrosis ( Fig. 3f ). First, fibrotic changes were already observed at an age of 3 weeks and steadily progressed over time. At the age of 12 weeks, the dermis was almost sixfold thicker in Wnt-10b tg mice than in control mice ( Fig. 3f ). The hydroxyproline content of the skin progressively increased in Wnt-10b tg mice and was tenfold higher in 12-week-old mice. Myofibroblast counts were significantly increased in Wnt-10b tg mice ( Fig. 3f ). To investigate whether pharmacological activation of the canonical Wnt pathway induces fibrosis, non-transgenic mice challenged with bleomycin were treated with R-spondin-1, a secreted protein that interacts with LRP6 and activates canonical Wnt signalling in the presence of Wnt ligands [32] , [33] , [34] . R-spondin-1 treatment augmented bleomycin-induced nuclear accumulation of β-catenin in fibroblasts and enhanced bleomycin-induced dermal fibrosis as shown by more severe dermal thickening, higher hydroxyproline content and increased myofibroblast counts ( Supplementary Fig. S4 ). Overexpression of Dkk-1 prevents fibrosis We next investigated whether inhibition of the canonical Wnt pathway blocks the development of fibrosis. Overexpression of the endogenous inhibitor Dkk-1 was chosen to target the canonical Wnt pathway, because Dkk-1 is downregulated in human and in experimental murine fibrosis and Dkk-1 is currently evaluated as a potential therapeutic target for other diseases [35] , [36] . We therefore interbred Wnt-10b tg mice with Dkk-1 tg mice to generate Wnt-10b/Dkk-1 double-mutant mice. Overexpression of Dkk-1 prevented the profibrotic effects of Wnt-10b on dermal thickening and normalized both hydroxyproline content and myofibroblast counts at 12 weeks to the levels of wild-type control mice ( Supplementary Fig. S5 ). Moreover, overexpression of Dkk-1 also protected from bleomycin-induced fibrosis. Bleomycin-induced dermal thickening, accumulation of hydroxyproline and myofibroblast differentiation was not observed in Dkk-1 tg mice ( Fig. 4a ). 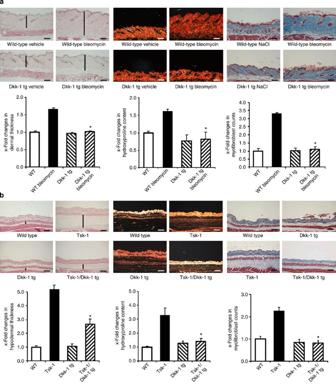Figure 4: Inhibition of canonical Wnt signalling by Dkk-1 prevents experimental fibrosis. (a) Dkk-1 transgenic (Dkk-1 tg) mice were resistant to bleomycin-induced fibrosis. Haematoxylin and eosin-, Sirius Red- and trichrome-stained sections are shown (horizontal scale bars, 100 μm). Challenge with bleomycin induced dermal fibrosis with increased dermal thickening, accumulation of hydroxyproline and myofibroblast differentiation in wild-type mice, but not in Dkk-1 tg littermates. In contrast to wild-type mice, these outcomes did not differ between Dkk-1 tg mice challenged with bleomycin and Dkk-1 tg mice injected with NaCl (n≥ 6 for all groups). (b) Dkk-1 prevented fibrosis in Tsk-1 mice. The histological changes induced by the Tsk-1 mutation in the fibrillin-1 gene are ameliorated by transgenic overexpression of Dkk-1, as shown in representative haematoxylin and eosin-, Sirius Red- and trichrome-stained sections (horizontal scale bars, 200 μm). Hypodermal thickening, hydroxyproline content and myofibroblast counts were all significantly reduced in Tsk-1/Dkk-1, as compared with Tsk-1 littermates not carrying the Dkk-1 transgene (n≥ 5 for all groups). Vertical black bars in these images indicate the dermal or hypodermal thickness. *IndicatesP-values of less than 0.05 as compared with wild-type mice challenged with bleomycin (a) and with Tsk-1 mice not transgenic for Dkk-1 (b), respectively, as analysed using the Mann–WhitneyU-test. All data are expressed as mean ± s.e.m. Figure 4: Inhibition of canonical Wnt signalling by Dkk-1 prevents experimental fibrosis. ( a ) Dkk-1 transgenic (Dkk-1 tg) mice were resistant to bleomycin-induced fibrosis. Haematoxylin and eosin-, Sirius Red- and trichrome-stained sections are shown (horizontal scale bars, 100 μm). Challenge with bleomycin induced dermal fibrosis with increased dermal thickening, accumulation of hydroxyproline and myofibroblast differentiation in wild-type mice, but not in Dkk-1 tg littermates. In contrast to wild-type mice, these outcomes did not differ between Dkk-1 tg mice challenged with bleomycin and Dkk-1 tg mice injected with NaCl ( n ≥ 6 for all groups). ( b ) Dkk-1 prevented fibrosis in Tsk-1 mice. The histological changes induced by the Tsk-1 mutation in the fibrillin-1 gene are ameliorated by transgenic overexpression of Dkk-1, as shown in representative haematoxylin and eosin-, Sirius Red- and trichrome-stained sections (horizontal scale bars, 200 μm). Hypodermal thickening, hydroxyproline content and myofibroblast counts were all significantly reduced in Tsk-1/Dkk-1, as compared with Tsk-1 littermates not carrying the Dkk-1 transgene ( n ≥ 5 for all groups). Vertical black bars in these images indicate the dermal or hypodermal thickness. *Indicates P -values of less than 0.05 as compared with wild-type mice challenged with bleomycin ( a ) and with Tsk-1 mice not transgenic for Dkk-1 ( b ), respectively, as analysed using the Mann–Whitney U -test. All data are expressed as mean ± s.e.m. Full size image To further substantiate the antifibrotic effect of Wnt blockade, we analysed whether overexpression of Dkk-1 ameliorates fibrosis in Tsk-1 mice. We therefore generated Dkk-1/Tsk-1 double-tg mice (Dkk-1/Tsk-1 mice) and compared fibrotic changes with those of Tsk-1 littermates. Fibrosis was significantly reduced in Dkk-1/Tsk-1 mice with reduced hypodermal thickening, hydroxyproline content and myofibroblast counts comparable with control mice not bearing the Tsk-1 mutation ( Fig. 4b ). We also performed loss-of-function studies using neutralizing antibodies against Dkk-1. Consistent with the finding that the levels of Dkk-1 are strongly decreased and almost undetectable in fibrotic diseases, neutralizing antibodies against Dkk-1 resulted only in a slight increase in fibrosis scores with nonsignificant increases in dermal thickness, myofibroblast counts and hydroxyproline content. However, treatment of Dkk-1 tg mice with neutralizing antibodies against Dkk-1 resulted in a significant exacerbation of fibrosis. The protective effects of the tg overexpression of Dkk-1 were almost completely abrogated by treatment with neutralizing antibodies against Dkk-1 ( Supplementary Fig. S6 ). To evaluate the effect of the neutralization of Dkk-1 in the absence of additional profibrotic stimuli, healthy mice were treated with neutralizing antibodies against Dkk-1. Although there was some trend, treatment of mice with neutralizing antibodies against Dkk-1 did not result in statistically significant increases in dermal thickness, number of myofibroblasts or hydroxyproline content compared with sham-treated control mice. We hypothesized that this may result from a counter-regulation in healthy mice that limits the activation of canonical Wnt signalling on neutralization of Dkk-1. Indeed, we observed only a slight increase in the number of fibroblasts with nuclear accumulation of β-catenin on treatment with neutralizing antibodies against Dkk-1 (24±3 versus 19±4 %). Consistently, the mRNA levels of axin-2 in the skin were also increased by only 26±9%. We also observed an increase of 97±12% in the mRNA levels of Dkk-2 in mice treated neutralizing antibodies against Dkk-1 compared with sham-treated controls. This compensatory increase of Dkk-2 did not occur under fibrotic conditions such as challenge with bleomycin or overexpression of TGF-β receptor (TBR). Thus, a compensatory increase in other endogenous inhibitors such as Dkk-2 may limit the activation of canonical Wnt signalling and prevents fibrosis on neutralization of Dkk-1 in healthy mice, whereas this escape mechanism is not operative in fibrotic conditions. TGF-β activates canonical Wnt signalling Because of the crucial role of TGF-β in fibrotic disease, we speculated that TGF-β signalling might contribute to activation of the canonical Wnt pathway. Stimulation with TGF-β induced nuclear accumulation of β-catenin in cultured fibroblasts ( Fig. 5a ) and increased the activity of Tcf/Lef-responsive elements in reporter assays ( Fig. 5b ). Moreover, the canonical Wnt pathway was activated in adenoviral overexpression of a constitutively active TGF-β receptor type I (Ad-TBRI act )-induced fibrosis with nuclear accumulation of β-catenin in fibroblasts and increased mRNA levels of axin-2 ( Fig. 5c and d ). 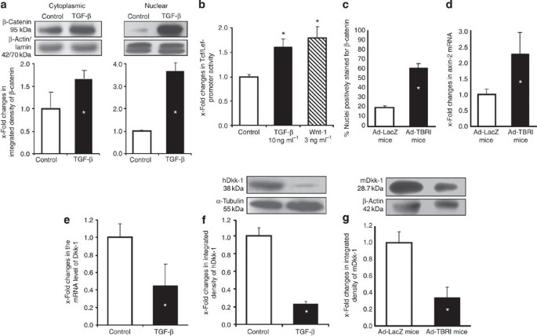Figure 5: TGF-β activates canonical Wnt signalling by decreasing Dkk-1. (a) TGF-β induces nuclear accumulation of β-catenin in cultured human fibroblasts as shown by Western blot from cytoplasmic and nuclear extracts (n=4). (b) TGF-β stimulates the activity of a TCF/Lef reporter construct (n=8). (c) Adenoviral overexpression of TBRIactin the skin of mice (Ad-TBRI) induced nuclear accumulation of β-catenin in fibroblasts as compared with control mice infected with adenovirus encoding for LacZ (Ad-LacZ) (n≥ 6). (d) Ad-TBRI uprgeulated the mRNA levels of the Wnt target gene axin-2 (n≥ 6). (e) Incubation with TGF-β reduced the mRNA levels of Dkk-1 in cultured fibroblasts (n=7). (f) TGF-β decreased the protein levels of Dkk-1 in cultured fibroblasts (n=5). (g) Decreased levels of Dkk-1 were also observed in the skin of Ad-TBRI mice by western blot (n=4). Representative bands and the mean results of the densiometric quantification are shown ina,fandg. * IndicatesP-values of less than 0.05 as compared with unstimulated cells (a,b,eandf, as analysed with the Wilcoxon signed-rank test) and with Ad-LacZ mice (c,dandg, as analysed using the Mann–WhitneyU-test). All data are expressed as mean ± s.e.m. Figure 5: TGF-β activates canonical Wnt signalling by decreasing Dkk-1. ( a ) TGF-β induces nuclear accumulation of β-catenin in cultured human fibroblasts as shown by Western blot from cytoplasmic and nuclear extracts ( n =4). ( b ) TGF-β stimulates the activity of a TCF/Lef reporter construct ( n =8). ( c ) Adenoviral overexpression of TBRI act in the skin of mice (Ad-TBRI) induced nuclear accumulation of β-catenin in fibroblasts as compared with control mice infected with adenovirus encoding for LacZ (Ad-LacZ) ( n ≥ 6). ( d ) Ad-TBRI uprgeulated the mRNA levels of the Wnt target gene axin-2 ( n ≥ 6). ( e ) Incubation with TGF-β reduced the mRNA levels of Dkk-1 in cultured fibroblasts ( n =7). ( f ) TGF-β decreased the protein levels of Dkk-1 in cultured fibroblasts ( n =5). ( g ) Decreased levels of Dkk-1 were also observed in the skin of Ad-TBRI mice by western blot ( n =4). Representative bands and the mean results of the densiometric quantification are shown in a , f and g . * Indicates P -values of less than 0.05 as compared with unstimulated cells ( a , b , e and f , as analysed with the Wilcoxon signed-rank test) and with Ad-LacZ mice ( c , d and g , as analysed using the Mann–Whitney U -test). All data are expressed as mean ± s.e.m. Full size image On the basis of the decreased expression of Dkk-1, we hypothesized that TGF-β signalling might regulate canonical Wnt signalling via Dkk-1. Stimulation with TGF-β reduced the levels of Dkk-1 mRNA and protein in dermal fibroblasts by 60 and 80%, respectively ( Fig. 5e and f ). Of note, we observed a decrease in Dkk-1 and an increase in TOP-reporter activity upon stimulation with TGF-β in human embryonic kidney 293 cells and in A549 pulmonary epithelial cells, indicating that the stimulatory effects of TGF-β on canonical Wnt signalling are not restricted to fibroblasts. Furthermore, overexpression of TBRI act in mice significantly reduced the expression of Dkk-1 ( Fig. 5g ). The TGF-β-mediated suppression of Dkk-1 was independent of the canonical Smad pathway, but was mediated by the mitogen-activated kinase p38. Short interfering RNA (siRNA) against Smad4 effectively reduced the levels of Smad4 and also decreased the expression of the Smad target plasminogen-activator inhibitor-1 in fibroblasts, but did not prevent the decrease of Dkk-1 mRNA and protein on incubation with TGF-β ( Supplementary Fig. S7a ). siRNA against Smad3 also did not prevent the inhibitory effects of TGF-β on Dkk-1. Using pharmacological inhibitors as well as siRNA, we demonstrated that p38 is crucial for the inhibitory effects of TGF-β on the expression of Dkk-1 ( Supplementary Fig. S7b and S7c ). Inhibition of p38 completely prevented the downregulation of Dkk-1 by TGF-β. In contrast, inhibition of Rock, JNK and Rac, all of which have been implicated in TGF-β signalling as well, did not reduce the inhibitory effects of TGF-β on the expression of Dkk-1 ( Supplementary Fig. S7b ). When fibroblasts were stimulated with TGF-β in the presence of recombinant Dkk-1, activation of canonical Wnt signalling was significantly reduced as shown by impaired nuclear accumulation of β-catenin ( Fig. 6a and b ) and activation of Tcf/Lef-responsive elements ( Fig. 6c ). Consistent with these in vitro results, tg overexpression of Dkk-1 prevented the Ad-TBRI act -induced activation of the canonical Wnt pathway in mice and reduced the nuclear accumulation of β-catenin in fibroblasts and mRNA levels of axin-2 to the levels of wild-type control mice ( Fig. 6d and e ). 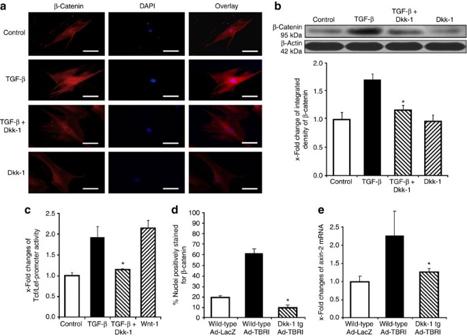Figure 6: Dkk-1 prevented the stimulatory effects of TGF-β on canonical Wnt signalling. (a) Recombinant Dkk-1 abrogated the TGF-β induced nuclear accumulation of β-catenin as assessed by immunofluorescence (n=6). (b) The inhibitory effects of Dkk-1 on the TGF-β-induced nuclear accumulation of β-catenin were confirmed by western blot (n=4). (c) Dkk-1 prevented the TGF-β-induced activation of a TCF/Lef reporter constructin vitro.Recombinant Wnt-1 was used as a positive control (n=8). (d) Nuclear accumulation of β-catenin was observed in wild-type mice infected with adenovirus encoding for TBRIact(Ad-TBR), but not in Dkk-1 transgenic mice (Dkk-1 tg;n≥ 5 for all groups). (e) Ad-TBRI increased the mRNA levels of axin-2 in wild-type mice, but not Dkk-1 tg mice (n≥ 5 for all groups). * IndicatesP-values of less than 0.05 as compared with cells stimulated with TGF-β (b,c) or with wild-type mice infected with Ad-TBRI (d,e). All results were analysed using the Wilcoxon signed-rank test. All data are expressed as mean ± s.e.m. Figure 6: Dkk-1 prevented the stimulatory effects of TGF-β on canonical Wnt signalling. ( a ) Recombinant Dkk-1 abrogated the TGF-β induced nuclear accumulation of β-catenin as assessed by immunofluorescence ( n =6). ( b ) The inhibitory effects of Dkk-1 on the TGF-β-induced nuclear accumulation of β-catenin were confirmed by western blot ( n =4). ( c ) Dkk-1 prevented the TGF-β-induced activation of a TCF/Lef reporter construct in vitro. Recombinant Wnt-1 was used as a positive control ( n =8). ( d ) Nuclear accumulation of β-catenin was observed in wild-type mice infected with adenovirus encoding for TBRI act (Ad-TBR), but not in Dkk-1 transgenic mice (Dkk-1 tg; n ≥ 5 for all groups). ( e ) Ad-TBRI increased the mRNA levels of axin-2 in wild-type mice, but not Dkk-1 tg mice ( n ≥ 5 for all groups). * Indicates P -values of less than 0.05 as compared with cells stimulated with TGF-β ( b , c ) or with wild-type mice infected with Ad-TBRI ( d , e ). All results were analysed using the Wilcoxon signed-rank test. All data are expressed as mean ± s.e.m. Full size image To confirm the importance of TGF-β for the activation of the canonical Wnt pathway in fibrosis, we also evaluated the effects of the selective TBRI inhibitor SD-208 on canonical Wnt signalling. Treatment with SD-208 significantly reduced the nuclear accumulation of β-catenin in activated fibroblasts and prevented the increase in axin-2 mRNA levels in bleomycin-induced fibrosis, Tsk-1 mice and Ad-TBRI act -induced fibrosis ( Fig. 7a and b ; Supplementary Fig. S8 ), highlighting that TGF-β has a key role for the activation of the canonical Wnt cascade in fibrosis. 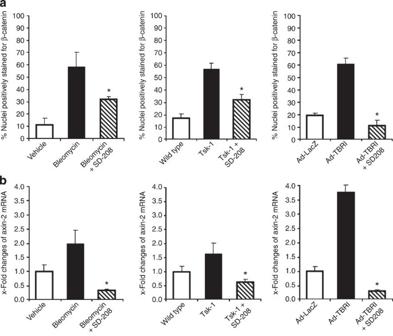Figure 7: Inhibition of TGF-β signalling reduces the activation of canonical Wnt in experimental fibrosis. (a) Treatment with SD-208, a selective inhibitor of TBRI, significantly decreased the nuclear accumulation of β-catenin in fibroblasts in bleomycin-induced dermal fibrosis, in Tsk-1 mice and in TBRIactinduced fibrosis (n≥ 5 for all groups in all models). (b) SD-208 completely prevented the increase in the mRNA levels of axin-2 in these mouse models (n≥ 5 for all groups in all models). * IndicatesP-values of less than 0.05 (as analysed with the Mann–WhitneyU-test) compared with bleomycin treated-, Tsk-1, or TBRIactmice without SD-208. All data are expressed as mean ± s.e.m. Figure 7: Inhibition of TGF-β signalling reduces the activation of canonical Wnt in experimental fibrosis. ( a ) Treatment with SD-208, a selective inhibitor of TBRI, significantly decreased the nuclear accumulation of β-catenin in fibroblasts in bleomycin-induced dermal fibrosis, in Tsk-1 mice and in TBRI act induced fibrosis ( n ≥ 5 for all groups in all models). ( b ) SD-208 completely prevented the increase in the mRNA levels of axin-2 in these mouse models ( n ≥ 5 for all groups in all models). * Indicates P -values of less than 0.05 (as analysed with the Mann–Whitney U -test) compared with bleomycin treated-, Tsk-1, or TBRI act mice without SD-208. All data are expressed as mean ± s.e.m. Full size image Dkk-1 ameliorates Ad-TBRI act -induced fibrosis To determine whether the downregulation of Dkk-1 is required for the profibrotic effects of TGF-β, we evaluated the extent of fibrosis in Dkk-1 tg mice infected with Ad-TBRI act . Overexpression of TBRI act in the skin induced dermal fibrosis in wild-type mice with dermal thickening, increased hydroxyproline content and myofibroblast differentiation as compared with control mice infected with Ad-LacZ. In contrast, Dkk-1 tg mice were protected from Ad-TBRI act -induced fibrosis. Dermal thickening, hydroxyproline content and myofibroblast counts on infection with Ad-TBRI act were significantly reduced in Dkk-1 tg mice as compared with wild-type littermates ( Fig. 8 ). These findings indicate that the regulation of Dkk-1 by TGF-β has an important role in the pathogenesis of fibrosis. 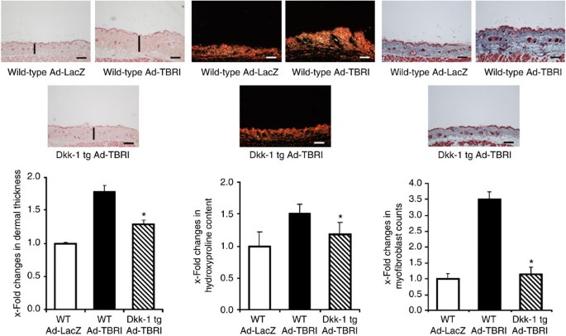Figure 8: Inhibition of canonical Wnt signalling by Dkk-1 prevents Ad-TBRIact-induced fibrosis. Intradermal infection with adenoviruses encoding for TBRIact(Ad-TBRI) induced dermal fibrosis in wild-type mice, but not in Dkk-1 transgenic (Dkk-1 tg) littermates. Representative histological sections stained with haematoxylin and eosin, Sirius Red and trichrome are shown (horizontal scale bar, 100 μm). The dermal thickening observed in wild-type mice on infection with Ad-TBRI was significantly ameliorated in Dkk-1 transgenic (Dkk-1 tg) mice. The Ad-TBRI-mediated increases in hydroxyproline content and in the number of myofibroblasts were also reduced in Dkk-1 tg mice (n≥ 5 for all groups). * IndicatesP-values of less than 0.05 (as analysed using the Mann–WhitneyU-test) compared with wild-type mice infected with Ad-TBRI. All data are expressed as mean ± s.e.m. Figure 8: Inhibition of canonical Wnt signalling by Dkk-1 prevents Ad-TBRI act -induced fibrosis. Intradermal infection with adenoviruses encoding for TBRI act (Ad-TBRI) induced dermal fibrosis in wild-type mice, but not in Dkk-1 transgenic (Dkk-1 tg) littermates. Representative histological sections stained with haematoxylin and eosin, Sirius Red and trichrome are shown (horizontal scale bar, 100 μm). The dermal thickening observed in wild-type mice on infection with Ad-TBRI was significantly ameliorated in Dkk-1 transgenic (Dkk-1 tg) mice. The Ad-TBRI-mediated increases in hydroxyproline content and in the number of myofibroblasts were also reduced in Dkk-1 tg mice ( n ≥ 5 for all groups). * Indicates P -values of less than 0.05 (as analysed using the Mann–Whitney U -test) compared with wild-type mice infected with Ad-TBRI. All data are expressed as mean ± s.e.m. Full size image Activation of the canonical Wnt pathway seems to be a general feature of fibrotic diseases that occurs in systemic fibrotic diseases such as SSc, but also in isolated organ fibrosis such as pulmonary, renal or liver fibrosis. Indeed, pathologically activated canonical Wnt signalling has been implicated in various fibrotic diseases [18] , [19] , [20] , [21] , [22] , [23] , [24] , [25] , [26] , [27] . We observed an overexpression of the Wnt proteins Wnt-1 and Wnt-10b in human samples from different fibrotic diseases and also a significantly decreased expression of the endogenous inhibitor Dkk-1. These changes resulted in an activation of the canonical Wnt pathway with nuclear accumulation of β-catenin and increased transcription of target genes in SSc, idiopathic pulmonary fibrosis and liver cirrhosis. The activation of the canonical Wnt pathway has a key role for fibroblast activation and collagen release in fibrosis. Wnt signalling stimulated the differentiation of resting fibroblasts into myofibroblasts, increased the release of extracellular matrix components and induced fibrosis. Of note, fibrotic disease induced by Wnt activation was more pronounced than the effects of other fibrotic pathways [37] . The activation of the canonical Wnt pathway and its potent profibrotic effects suggest that the Wnt pathway might be a potential target for novel antifibrotic approaches. We have chosen overexpression of the endogenous inhibitor Dkk-1 to inhibit the canonical Wnt pathway, because, first, decreased levels of Dkk-1 contributed to the activation of the canonical Wnt pathway in human fibrosis, second, Dkk-1 is currently investigated as a potential therapeutic target in other diseases [35] , [36] and third, this approach allows broader inhibition of the canonical Wnt pathway than targeting single Wnt proteins. Overexpression of Dkk-1 prevented fibrosis in inflammation-driven models such as the bleomycin model as well as in inflammation-independent models such as fibrosis in Tsk-1 mice, indicating that inhibition of the canonical Wnt pathway might be effective in acute as well as in chronic stages of fibrotic disease. Of particular interest, our data highlight the crosstalk between TGF-β signalling and the canonical Wnt pathway. Activated TGF-β signalling is a common denominator of fibrotic diseases [5] . We demonstrate on multiple experimental levels that TGF-β activates the canonical Wnt pathway. TGF-β seems to be the major stimulus for the activation of the canonical Wnt pathway in fibrotic diseases, because inhibition of TGF-β signalling by a selective TBRI inhibitor strongly reduced the activation of the canonical Wnt pathway in experimental fibrosis. We identified TGF-β-mediated decrease of Dkk-1 via p38 as major molecular mechanism for the activation of the canonical Wnt pathway. Furthermore, addition of recombinant Dkk-1 abrogated the stimulatory effects of TGF-β on the canonical Wnt pathway in fibroblasts. However, in other cell types, TGF-β might also stimulate Wnt signalling by other mechanisms such as inhibition of Glycogen Synthase Kinase-3β aside decreasing Dkk-1 (refs 38 , 39 ). Although the TGF-β-induced repression of Dkk-1 was independent of Smad3 and Smad4, our findings do not exclude a role of Smad proteins in the regulation of canonical Wnt signalling, as overexpression of Smad3 stimulated TOPflash reporter activity independent of TGF-β [40] . TGF-β activates a plethora of intracellular signalling cascades [41] . However, the molecular mediators of the profibrotic effects of TGF-β are only partially understood and the best targets for antifibrotic therapies have not yet been identified. Although the key role of TGF-β signalling for fibrosis is undoubted, first attempts to target TGF-β signalling in humans failed. CAT-192, a neutralizing antibody against TGF-β1, was ineffective due to low-affinity binding of TGF-β1 (ref. 42 ). Targeting the downstream mediator c-Abl in combination with platelet-derived growth factor receptor also did not yield major benefits [43] . Inhibition of the canonical Wnt pathway might be a novel approach to prevent the profibrotic effects of TGF-β signalling. Our data implicate that interaction of the canonical Wnt pathway and TGF-β is an important mechanism for fibrotic diseases. Inhibition of this pathway by Dkk-1 significantly reduced the stimulatory effects of TGF-β on fibroblasts and prevented Ad-TBRI act -induced fibrosis. Notably, TGF-β also has a major role in bleomycin-induced fibrosis and particularly Tsk-1 mice, which showed reduced fibrosis in Dkk-1 tg animals. Together, these data indicate that inhibition of the canonical Wnt pathway might be an effective approach to target TGF-β signalling in fibrotic diseases. Patients Skin biopsies were obtained from 12 SSc patients and ten age- and sex-matched healthy volunteers. All patients fulfilled the criteria for SSc, as suggested by LeRoy and Medsger [44] . Ten patients were women, and two were men. The age ranged from 30 to 51 years (median 38 years). All patients had diffuse cutaneous SSc. Lung tissue was obtained from eight patients with IPF and six matched non-fibrotic controls obtained from patients who died from head trauma (3) and from patients who had biopsy for suspected lung metastasis of different tumours (3). Of the patients with IPF, five were women and three were men. The age ranged from 42 to 72 years (median 54 years). Liver samples were obtained from five patients with alcoholic liver cirrhosis and five controls who died from head trauma (3) and from patients who had biopsy for suspected liver metastasis (2). Two of the patients with liver cirrhosis were women and three were men. The age ranged from 38 to 68 years (median 50 years). All samples from trauma patients were obtained within 3 h after the diagnosis of death. All biopsies taken for suspected metastasis were judged to be tumour-free by two independent pathologists. The human studies were approved by the Ethical committee of the Medical faculty of the University of Erlangen-Nuremberg. Cell culture Human fibroblasts were prepared as outgrowth cultures from eight skin biopsies and cultured as described [45] . In selected experiments, fibroblasts were stimulated with recombinant TGF-β (10 ng ml −1 ; R&D Systems, Ambington, UK) and recombinant human Wnt-1 (0.3–3 ng ml −1 ; PeproTech, Hamburg, Germany). Stimulation experiments were performed in DMEM/0.1% FCS. Fibroblasts from passages four to eight were used for the experiments. All patients and controls signed a consent form approved by the local institutional review board. Animals and treatments Mice overexpressing Wnt-10b under the FABP4 promoter (Wnt-10b tg mice) and Dkk-1 under the Col1a1 2.3-kb promoter (DKK1 tg mice) have previously been described [46] , [47] . The role of the Wnt cascade for fibrosis was investigated in three different models. (i) In the bleomycin-induced fibrosis model, dermal fibrosis was induced in six-week-old mice by repeated subcutaneous injections of 100 μl of bleomycin at a concentration of 0.5 mg ml −1 into defined areas of 1 cm 2 at the upper back every other day for 4 weeks [48] . Mice challenged with 0.9% NaCl served as controls. (ii) In the Tsk-1 model, a dominant mutation of the fibrillin-1 gene activates profibrotic signalling cascades and induces a SSc-like phenotype in fibroblasts with endogenous activation, and persistently increased release of collagen [49] . Tsk-1 mice are characterized by progressive accumulation of collagen and hypodermal thickening. (iii) Ad-TBRI act (refs 50 , 51 ) served as a model of TGF-β signalling-mediated fibrosis. Replication-deficient type 5 adenoviruses encoding for TBRI act or LacZ were injected at concentrations of 6.7×10 7 p.f.u. per mouse into defined areas of 1 cm 2 at the upper back. The first injection was performed at an age of 4 weeks and repeated 4 weeks later. The mice were killed 4 weeks after the last injection. To maximally activate the Wnt cascade in vivo , mice were treated with the Wnt-agonist R-spondin (kindly provided by A. Arbo). Recombinant R-spondin was injected subcutaneously at a concentration of 8 mg per kg per day for 4 weeks. Neutralizing antibodies against murine Dkk-1 were kindly provided by W. Richards. Rat anti-Dkk-1 antibodies were administered by intraperitoneal injections three times per week at a dose of 50 mg kg −1 as described [52] . For selective inhibition of TGF-β signalling, mice were treated with SD-208 at doses of 20 mg kg −1 orally. SD-208 is an active ATP-competitive inhibitor of TBRI with an IC 50 of 49 nM, which displays a >100-fold and a >17-fold selectivity over TGF-βRII and other common kinases, respectively [53] . All mouse experiments were approved by the government of Mittelfranken. Reporter assays A Col1a2 promoter–luciferase construct containing the fragment between −353 and +58 nucleotides of Col1a2 was kindly provided by M. Trojanowska [54] . TOP Flash plasmids and FOP Flash plasmids containing three wild-type or three mutated copies of Tcf consensus binding sites upstream of firefly luciferase complementary DNA were purchased from Millipore Corporation (Billerica, MA, USA). A common β-galactosidase reporter vector (Sigma-Aldrich, Steinheim, Germany) was used as control. Luciferase and β-galactosidase activities were determined using a microplate luminometer (Berthold Technologies, Bad Herrenalb, Germany) and a MRX ELISA reader (Dynex Technologies, Chantilly, USA). Quantitative real-time PCR Gene expression was quantified by TaqMan and SYBR Green real-time PCR using the ABI Prism 7300 Sequence Detection System (Applied Biosystems, Foster City, CA, USA) [55] . Specific primer pairs for each gene were designed with the Primer 3 software. The following primer pairs were used: human axin-2: 5′-CATGACGGACAGCAGTGTAGA-3′ (forward), 5′-TACTGCCCACACGATAAGGAG-3′ (reverse); murine axin-2: 5′-GCCACCAAGACCTACATACGA-3′ (forward), 5′-GAGCCGATCTGTTGCTTCTT-3′ (reverse); human Dkk-1: 5′-GACTGTGCCTCAGGATTGTGT-3′ (forward), 5′-CAGATCTTGGACCAGAAGTGTCT-3′ (reverse); human α1(I) procollagen: 5′-TCAAGAGAAGGCTCACGATGG-3′ (forward), 5′-TCACGGTCACGAACCACATT-3′ (reverse); human αSMA: 5′-AAGAGGAATCCTGACCCTGAA-3′ (forward), 5′-TGGTGATGATGCCATGTTCT-3′ (reverse); murine αSMA: 5′-ATGCCTCTGGACGTACAACTG-3′ (forward), 5′-CACACCATCTCCAGAGTCCA-3′ (reverse). Samples without enzyme in the reverse transcription reaction (Non-RT controls) were used as negative controls. Unspecific signals caused by primer dimers were excluded by no template controls and by dissociation curve analysis. A predeveloped β-actin assay (Applied Biosystems) was used to normalize for the amounts of cDNA within each sample. Quantification of collagen protein The amount of soluble collagen in cell culture supernatants was quantified using the SirCol collagen assay (Biocolor, Belfast, Northern Ireland) [56] . The total collagen content in skin samples including insoluble collagen was determined by hydroxyproline assays [57] . Visualization of stress fibres Actin stress fibres were visualized with rhodamine-conjugated phalloidin (Molecular Probes, Eugene, OR, USA) [56] and analysed using a Nikon Eclipse 80i microscope (Nikon, Badhoevedorp, The Netherlands). Western blot analysis Western blotting was performed using monoclonal antibodies against αSMA (Sigma-Aldrich), polyclonal anti-Dkk-1 antibodies (R&D Systems), anti-β-catenin (R&D Systems), anti-Smad3 and anti-Smad4 (Santa Cruz Biotechnology, Heidelberg, Germany) and anti-p38 (Cell Signaling Technology, Danvers, MA, USA). Equal loading of proteins was confirmed by visualization of α-tubulin (Invitrogen, Darmstadt, Germany) or β-actin (Sigma-Aldrich). The western blot bands were quantified using ImageJ Software (version 1.41). siRNA-mediated gene silencing Fibroblasts were transfected with 1.5-μg siRNA reagent (ON-TARGET plus smart pool) for human Smad3 and Smad4 or prevalidated siRNAs against p38α, p38β, p38γ and p38δ (all Dharmacon, Lafayette, CO, USA) using the human fibroblast Nucleofector kit (Amaxa GmbH, Cologne, Germany). Fibroblasts transfected with non-targeting control siRNAs (Ambion, Darmstadt, Germany) were used as controls. Medium was changed after 6 h to remove the nucleofector solution. Cells were collected for further analyses after 36 h. Pharmacologic inhibition of TGF-β-dependent pathways To inhibit non-canonical, Smad-independent intracellular TGF-β pathways, fibroblasts were incubated with the Rock inhibitor Y27632 (1 μM, Calbiochem, Darmstadt, Germany), the p38 inhibitor SB202190 (10 μM, Tocris Bioscience, Bristol, UK), the JNK inhibitor SP600125 (1 μM, Tocris Bioscience) and the Rac inhibitor NSC23766 (300 μM, Tocris Bioscience). Histology Paraffin-embedded tissue sections were stained with haematoxylin and eosin, with trichrome or with Sirius Red, according to common protocols [58] . The dermal thickness was analysed with a Nikon Eclipse 80i microscope (Nikon) by measuring the maximal distance between the epidermal–dermal junction and the dermal–subcutaneous fat junction at four different skin sections of each mouse as described [48] . The hypodermal thickness was determined by measuring the thickness of the subcutaneous connective tissue beneath the panniculus carnosus at four different sites at the upper back in each mouse. The evaluation was performed by two independent, blinded examiners. Immunohistochemistry and confocal microscopy Formalin-fixed, paraffin-embedded skin sections were stained with anti-β-catenin antibodies (R&D Systems), anti-αSMA antibodies (Sigma-Aldrich), anti-Wnt-1 antibodies (Abcam, Cambridge, UK), anti-Wnt-10b antibodies (ProSci Incorporated, Poway, CA, USA), anti-murine Dkk-1 (R&D Systems) and anti-human Dkk-1 (R&D Systems). Concentration-matched species-specific immunoglobulins (Vector, Burlingame, CA, USA) were used as control antibodies. Biotinylated secondary antibodies and fluorescence-labelled streptavidin complexes (CF488A or CF594) (all Vector) were used for visualization. To identify nuclear accumulation of β-catenin in fibroblasts, skin sections were triple stained for β-catenin, DAPI and either the fibroblast markers prolyl-4-hydroxylase-β (Acris Antibodies, Herford, Germany) or vimentin (Sigma-Aldrich) or the myofibroblast marker αSMA. In addition, costainings for β-catenin, the epithelial marker E-cadherin (Dako, Glostrup, Denmark) and DAPI were performed. Confocal images were obtained by using a LSM 700 microscope (Carl Zeiss, Jena, Germany) at 594 and 488 nm. For quantification of myofibroblasts, single, spindle-shaped cells in the dermis positive for αSMA were counted in six randomly chosen high-power fields at 200-fold magnification by two experienced researchers in a blinded manner as described [48] , [56] , [58] . Statistical analysis Data are expressed as mean±s.e.m. The Wilcoxon signed-rank tests for related samples and the Mann–Whitney U -test for non-related samples were used for statistical analyses. In a subset of experiments, the mean values of the control groups were set to 1. All other values were expressed as x-fold changes compared with the respective controls used as 'comparison mean values'. P -values <0.05 were considered statistically significant. How to cite this article: Akhmetshina, A. et al . Activation of canonical Wnt signalling is required for TGF-β-mediated fibrosis. Nat. Commun. 3:735 doi: 10.1038/ncomms1734 (2012).